Marine sequestration of carbon in bacterial metabolites Linking microbial metabolomics and carbon sequestration in the ocean via refractory organic molecules has been hampered by the chemical complexity of dissolved organic matter (DOM). Here, using bioassay experiments and ultra-high resolution metabolic profiling, we demonstrate that marine bacteria rapidly utilize simple organic molecules and produce exometabolites of remarkable molecular and structural diversity. Bacterial DOM is similar in chemical composition and structural complexity to naturally occurring DOM in sea water. An appreciable fraction of bacterial DOM has molecular and structural properties that are consistent with those of refractory molecules in the ocean, indicating a dominant role for bacteria in shaping the refractory nature of marine DOM. The rapid production of chemically complex and persistent molecules from simple biochemicals demonstrates a positive feedback between primary production and refractory DOM formation. It appears that carbon sequestration in diverse and structurally complex dissolved molecules that persist in the environment is largely driven by bacteria. Dissolved organic matter (DOM) in the ocean is a large reservoir of reduced carbon (662 Pg C) that is linked to atmospheric CO 2 through the biological processes of photosynthesis and respiration [1] . Microorganisms are the most abundant producers and consumers of marine organic matter, with bacteria playing a dominant role in the consumption and alteration of DOM [2] . The chemical composition and biological reactivity of DOM are modified during microbial utilization and processing, resulting in small dissolved molecules (<10 kDa) that are very resistant to further microbial alteration and consumption [3] . Microbial production of this refractory DOM contributes substantially to carbon sequestration in the ocean, a process recently termed the microbial carbon pump [3] , [4] . Refractory DOM in the ocean is on average 4,000–6,000 years old [5] , represents >90% of the total dissolved organic carbon reservoir and has a production rate of 43 Tg C per year [6] . The chemical complexity and refractory nature of DOM is enigmatic, and mechanistic interpretations of these properties often invoke abiotic reactions [7] . Many studies address the extensive metabolic potential of marine bacteria and archaea [8] , [9] , but the chemical complexity of bacterially produced dissolved organic molecules and its implications for the global carbon cycle is not well constrained. Complexity is a common property of natural organic mixtures and can be divided into compositional and structural diversity. Here compositional diversity refers to the number of different combinations of atoms as molecules in a mixture, whereas the vastly more expansive structural diversity refers to the chemically feasible arrangements of atoms in molecular environments, like functional groups and isomers. The chemical complexity of bacterial DOM was investigated using bioassay experiments conducted in the dark (21–26 °C) with a coastal seawater microbial inoculum and two different substrate amendments. A natural microbial assemblage (<1.5 μm pore size) was added (1:840 v/v) to large volume incubations with artificial sea water (42 l) and either glucose and glutamic acid (283 μM C, ‘monomers’) or a mixture of oligosaccharides and oligopeptides (269 μM C, ‘oligomers’) as sole carbon sources. Inorganic nutrients (nitrate and phosphate) were added to establish an initial molar ratio of 106C:16N:1P in the incubations. The abundance of bacteria and nanoflagellates during the incubations were determined by epifluorescence microscopy [10] , concentrations of total and dissolved organic carbon were determined by high-temperature combustion [10] and dissolved hydrolysable amino acids were determined by high-performance liquid chromatography [11] . At the end of the 29-day incubations, DOM was isolated by solid-phase extraction (SPE) and analysed by Fourier transform ion cyclotron resonance mass spectrometry [12] and high-field nuclear magnetic resonance spectroscopy (NMR) [13] . These complementary untargeted analyses provide novel insights into the biological generation of chemical complexity and the molecular imprint of microbes on DOM in the ocean. DOM production by a coastal bacterial inoculum The monomer substrates were rapidly (1.5 days) respired, incorporated into bacterial biomass or released as dissolved molecules ( Fig. 1a ). Bacterial abundance increased exponentially and peaked at 1.2 × 10 10 cells l −1 on day 3 ( Fig. 1c ). Following an initial lag phase of 1.5 days, the oligomer substrates also supported high bacterial growth (1.1 × 10 10 cells l −1 on day 5, Fig. 1b,d ). Bacteria rapidly released exometabolites during the utilization of the substrates, as indicated by the accumulation of dissolved organic carbon and total dissolved amino acids during the first 4–7 days, before the measurable appearance of nanoflagellate grazers ( Fig. 1a–f ). The high D/L ratios of the enantiomers of amino acids are a clear indication of the bacterial origin of the exometabolites in the bioassays ( Fig. 1e,f ). The net release of dissolved organic carbon on day 10 in both experiments corresponded with sharp declines in bacterial abundance and increases in nanoflagellate abundance and is attributed to grazing. The DOM released during grazing was rich in bacterial metabolites, as indicated by an increase in the D/L ratio of amino acid enantiomers ( Fig. 1e,f ). Nanoflagellate grazers and bacteriophage enhance particulate to dissolved organic matter transitions and carbon remineralization processes, thereby contributing to the chemical diversity of DOM [14] , [15] , [16] . Microbial population dynamics and organic carbon concentrations were reaching stable conditions by the end of the bioassays. Dissolved organic carbon concentrations were 10 and 11 μmol C l −1 , about 5% of the added organic carbon as observed in other long-time bioassays [3] , [17] . Most of the DOM that persisted until the end of the experiment was directly or indirectly released from bacteria, as indicated by significantly higher D/L ratios of amino acid enantiomers as compared with the ratio in intact bacterial cells ( Fig. 1e,f ). 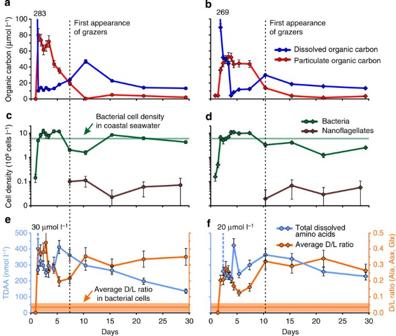Figure 1: Bioassay experiments with a coastal microbial inoculum. Dissolved (blue) and particulate organic carbon (red) concentrations (a,b) and bacterial (green) and heterotrophic nanoflagellate (brown) cell densities (c,d, log10scale) in the two bioassays amended with monomer (left, circles) and oligomer (right, diamonds) substrates. Total dissolved hydrolysable amino acid concentration (TDAA, light blue) and the average D/L ratio (orange) of the three dominantD-amino acids in total DOM (e,f): Alanine (Ala), aspartic acid+asparagine (Asx) and glutamic acid+glutamine (Glx). Both substrates only containedL-amino acids (30 and 20 μmol l−1, dashed light blue lines). Bacterial cell density in the coastal seawater (green bar) and the average D/L ratio (orange bar: 0.04±0.02 for Ala, Asx and Glx) in five representative marine bacterial cultures (data from ref.24) are shown for reference. The first appearance of nanoflagellates in epifluorescence microscopy samples is indicated by a black dashed line. Error bars are one s.d. and can be smaller than the symbol size. Figure 1: Bioassay experiments with a coastal microbial inoculum. Dissolved (blue) and particulate organic carbon (red) concentrations ( a , b ) and bacterial (green) and heterotrophic nanoflagellate (brown) cell densities ( c , d , log 10 scale) in the two bioassays amended with monomer (left, circles) and oligomer (right, diamonds) substrates. Total dissolved hydrolysable amino acid concentration (TDAA, light blue) and the average D/L ratio (orange) of the three dominant D -amino acids in total DOM ( e , f ): Alanine (Ala), aspartic acid+asparagine (Asx) and glutamic acid+glutamine (Glx). Both substrates only contained L -amino acids (30 and 20 μmol l −1 , dashed light blue lines). Bacterial cell density in the coastal seawater (green bar) and the average D/L ratio (orange bar: 0.04±0.02 for Ala, Asx and Glx) in five representative marine bacterial cultures (data from ref. 24 ) are shown for reference. The first appearance of nanoflagellates in epifluorescence microscopy samples is indicated by a black dashed line. Error bars are one s.d. and can be smaller than the symbol size. Full size image Molecular diversity of bacterial DOM The molecular and compositional diversity of DOM produced in the bioassay experiments was revealed by ultra-high resolution mass spectrometry. Molecular formulas were assigned to 1,720–1,800 mass peaks in the DOM extracted from the bioassays after 29 days. The DOM in both experiments consisted of molecules with similar molecular compositions and of comparable ranges of oxygen-to-carbon and hydrogen-to-carbon elemental ratios ( Fig. 2a,b ). About 50–60% of the molecular formulas in bacterial DOM were also present in coastal seawater DOM, representing 63–76% of the total spectral intensities of bacterial DOM ( Supplementary Fig. 1 ). Most (49–52%) of the molecules in bacterial DOM consisted solely of carbon, hydrogen and oxygen, whereas molecules containing nitrogen contributed 31–37% of the molecules ( Fig. 2c ). 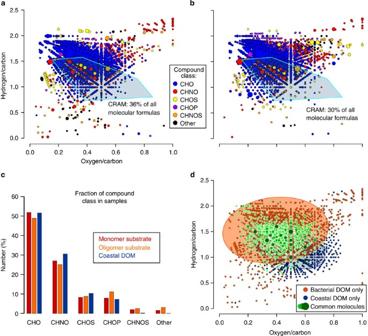Figure 2: The compositional diversity of bacterial DOM after 29 days. (a,b) Molecular formulas (MF) of bacterial DOM (monomer:a; and oligomer substrate:b) with compound classes (colours) and relative intensity (circle size) of the corresponding mass peaks. Data are displayed as molecular hydrogen-to-carbon versus oxygen-to-carbon ratio. Carboxyl-rich alicyclic molecules (CRAM) are located within the blue polygons. (c,d) Comparison of bacterial DOM with coastal DOM. (c) Number fraction of molecule compound classes highlight the compositional similarities among samples. (d) MF only present in combined bacterial DOM (red, 95% of total spectrum intensity focused in red shaded area), only in coastal DOM (blue, with 95% intensity area) and common MF in all samples (green, size and hue indicate number (maximum: 7) of superimposed MF per data point). Figure 2: The compositional diversity of bacterial DOM after 29 days. ( a , b ) Molecular formulas (MF) of bacterial DOM (monomer: a ; and oligomer substrate: b ) with compound classes (colours) and relative intensity (circle size) of the corresponding mass peaks. Data are displayed as molecular hydrogen-to-carbon versus oxygen-to-carbon ratio. Carboxyl-rich alicyclic molecules (CRAM) are located within the blue polygons. ( c , d ) Comparison of bacterial DOM with coastal DOM. ( c ) Number fraction of molecule compound classes highlight the compositional similarities among samples. ( d ) MF only present in combined bacterial DOM (red, 95% of total spectrum intensity focused in red shaded area), only in coastal DOM (blue, with 95% intensity area) and common MF in all samples (green, size and hue indicate number (maximum: 7) of superimposed MF per data point). Full size image Carboxyl-rich alicyclic molecules (CRAM) accounted for 30–36% of all bacterial DOM molecules in the bioassays and represented 30–34% of carboxyl-rich alicyclic molecules in the coastal seawater DOM ( Fig. 2 ). CRAM are a class of potentially refractory compounds identified in DOM from various aquatic environments [18] , [19] and represent a major fraction (>50%) of the molecular diversity in surface and deep-ocean DOM [13] . Bacteria also produced a suite of dissolved molecules ( n =116–144), which were identified previously as refractory components in the deep Atlantic Ocean with residence times greatly exceeding the oceanic mixing time [20] . On average, bacterial DOM was more saturated, less oxygenated and had a greater abundance of molecules with heteroatoms (P, N+S) compared with coastal seawater DOM ( Fig. 2c ). These observations point to a fraction of DOM potentially degradable on longer time scales and are consistent with other bioassay studies [17] , [21] . Long-term degradation of bacterial DOM under natural conditions decreases the average saturation and molecular mass of marine DOM molecules as shown for the Atlantic Ocean [22] . Overall, the similarities in elemental compositions and common molecules in bacterial and coastal seawater DOM ( Fig. 2c,d ) highlight the rapid generation of molecular diversity and potentially refractory molecules by bacterial metabolism. Structural diversity of bacterial DOM The structural diversity in the bacterial DOM produced in both bioassays was revealed by one- and two-dimensional NMR spectroscopy. The great diversity of functional groups and molecular environments resulted in mostly unresolved broad resonances in the proton and carbon spectra ( Fig. 3a,b ). The pronounced downfield shift of methyl and methylene proton resonances indicated spatial proximity of carbonyl derivatives, a characteristic of carboxyl-rich alicyclic molecules ( Fig. 4 ) [18] . The high ratio of carboxyl to aliphatic carbon (COO/CCH: 0.22–0.26) is compelling evidence for this structurally diverse group of apparently refractory molecules in bacterial DOM. Accordingly, carboxyl-rich alicyclic molecules accounted for up to 32–35% of the carbon in bacterial DOM (COO+CCH; Fig. 3b ) with protein and peptide amide carbon being a relatively minor component. Whether carboxyl-rich alicyclic molecules in the bioassays are structurally identical with those identified in the ocean remains to be elucidated. Bacterial secondary metabolites containing aromatic moieties are common [23] and the production of similar molecules in the bioassay experiments was apparent from a relatively high abundance and broad distribution of aromatic carbon ( Fig. 3b ). 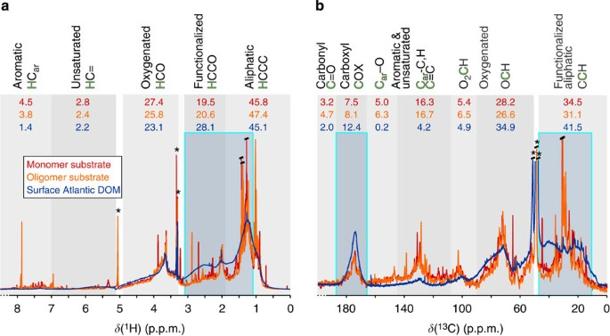Figure 3: The structural composition of bacterial after 29 days and open-ocean DOM. Proton (a) and carbon (b) NMR spectra of bacterial DOM with monomer (red) and oligomer (orange) substrate amendments and surface DOM (48 m depth) from the Atlantic Ocean (blue; cf. Figs 2 and 3 in ref.13) with general structural assignments (top). Relative proton and carbon fractions of key chemical environments were calculated from total NMR integrals (below; solvent peaks (*) excluded). Prominent peaks from high-abundance compounds in bacterial DOM contribute little to the total integrals and signal overlap. Major molecular features representing refractory carboyxl-rich alicyclic molecules (CRAM) are indicated by blue boxes. Figure 3: The structural composition of bacterial after 29 days and open-ocean DOM. Proton ( a ) and carbon ( b ) NMR spectra of bacterial DOM with monomer (red) and oligomer (orange) substrate amendments and surface DOM (48 m depth) from the Atlantic Ocean (blue; cf. Figs 2 and 3 in ref. 13 ) with general structural assignments (top). Relative proton and carbon fractions of key chemical environments were calculated from total NMR integrals (below; solvent peaks (*) excluded). Prominent peaks from high-abundance compounds in bacterial DOM contribute little to the total integrals and signal overlap. Major molecular features representing refractory carboyxl-rich alicyclic molecules (CRAM) are indicated by blue boxes. 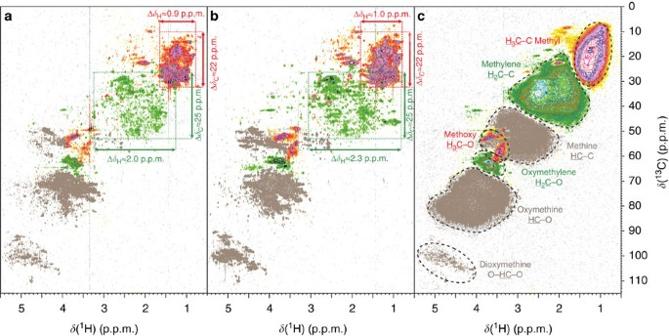Figure 4: The structural diversity of bacterial after 29 days and open-ocean DOM. 1H,13C–DEPT–HSQC–NMR spectra of the aliphatic region showing proton and carbon chemical shifts. Bacterial DOM from monomer (a) and oligomer (b) bioassay experiment and surface DOM (48 m depth) from the Atlantic Ocean (c; cf. Figs 7 and 8 in ref.13) are coloured according to methyl (CH3, red), methylene (CH2, green) and methine (CH, brown) carbon. The structural diversity of the bacterial DOM is apparent from the broad chemical shift ranges of the different carbon types (CH3: Δδ(1H)≈1 p.p.m.; Δδ(13C)≈22 p.p.m.; CH2: Δδ(1H)≈2 p.p.m.; and Δδ(13C)≈25 p.p.m.), in concurrence with the compositional diversity (Fig. 2). Open ocean-surface DOM (c) represents one of the most complex natural organic matter mixtures, delimiting the maximum chemically feasible ranges for molecular environments of each carbon type. Full size image Figure 4: The structural diversity of bacterial after 29 days and open-ocean DOM. 1 H, 13 C–DEPT–HSQC–NMR spectra of the aliphatic region showing proton and carbon chemical shifts. Bacterial DOM from monomer ( a ) and oligomer ( b ) bioassay experiment and surface DOM (48 m depth) from the Atlantic Ocean ( c ; cf. Figs 7 and 8 in ref. 13 ) are coloured according to methyl (CH 3 , red), methylene (CH 2 , green) and methine (CH, brown) carbon. The structural diversity of the bacterial DOM is apparent from the broad chemical shift ranges of the different carbon types (CH 3 : Δ δ ( 1 H)≈1 p.p.m. ; Δ δ ( 13 C)≈22 p.p.m. ; CH 2 : Δ δ ( 1 H)≈2 p.p.m. ; and Δ δ ( 13 C)≈25 p.p.m. ), in concurrence with the compositional diversity ( Fig. 2 ). Open ocean-surface DOM ( c ) represents one of the most complex natural organic matter mixtures, delimiting the maximum chemically feasible ranges for molecular environments of each carbon type. Full size image The chemical complexity of bacterial DOM was compared with DOM isolated from the surface Atlantic Ocean and analysed under the same experimental conditions [13] . Surface Atlantic DOM is dominated by refractory molecules that exist in an extremely complex mixture and is characterized by a smooth distribution of NMR resonances from extensive signal overlap [13] . The structural diversity of molecular environments in bacterial DOM was similar to that in Atlantic DOM, as indicated by the broad and congruent distribution of proton and carbon peaks in the one- and two-dimensional NMR spectra ( Figs 3 and 4 ). Bacterial DOM did not reflect the same extent of structural space coverage as surface Atlantic DOM ( Fig. 4c ), but the chemical complexity generated by bacterial metabolism provides novel insights about the mechanisms shaping the complexity of DOM. The bacterial imprint on the oceanic reservoir of DOM is readily apparent in the occurrence of a variety of biomarker compounds in sea water [24] , [25] , but the recognition that bacteria also shape the chemical complexity of DOM is surprising and alters our perception of the cycling of this globally significant carbon reservoir. Structural similarities between soil organic matter and microbially derived molecules have also been observed [26] , [27] . Given the ubiquitous distribution of microorganisms on Earth [28] , it appears much of the chemical complexity of natural organic matter in the biosphere is of microbial origin. This contrasts with the perception that the chemical complexity of natural organic matter is predominantly generated over long periods of time by abiotic processes. The rapid generation of a diverse and structurally complex mixture of molecules in these simple bioassay experiments is an expression of the integrated metabolic potential of the natural microbial community in a few millilitres of coastal sea water. Recent metabolic profiling studies also point to a perplexingly diverse microbial exometabolome [29] , [30] , [31] . Exometabolites play important roles in the organization of ecosystems and their functional roles include cell-to-cell signalling, iron acquisition and interspecies interactions [32] , [33] , [34] . The diversity of metabolites currently identified in microorganisms is small as compared with the extensive putative biosynthetic pathways suggested from whole or community genome sequencing [35] , [36] . Microbial growth dynamics varied initially between substrates in the experiments and differences in the structural and compositional features of bacterial DOM were observed. The reasons for these differences are not apparent but could reflect varying microbial diversity, cell differentiation and metabolite exchange promoted by the different substrates. We now face the challenge of understanding the unknown functional roles of potentially tens of thousands of exometabolites and how they might persist in the ocean. The dissolved organic carbon concentrations at the end of the bioassays (≈10 μmol l −1 ) are about four times lower than those in the deep ocean. This carbon is divided among thousands of molecular formulas and an untold number of isomers, indicating the concentrations of individual molecules are extremely low and potentially limiting for bacterial transport and utilization [37] , [38] . Some of the bacterial DOM accumulated after 29 days would likely be consumed or transformed under different conditions, yet the chemical complexity and refractory character of DOM that were initially established would persist [3] , [17] . The structural complexity of DOM places profound constraints on bacterial transport and utilization. A myriad of transporter proteins and catabolic enzymes would be required for the utilization of such a structural potpourri of substrates. The diversity of active bacteria in the ocean is high [39] , but the metabolic potential for utilizing the vast range of substrates is not uniformly distributed [35] , [40] , further reducing encounter rates between substrates and enzymes. Physicochemical associations of molecules, low metabolic energy yields and environmental conditions can also limit the microbial utilization of DOM [7] , [37] , [41] . Global ocean primary production rivals that on land [42] . The sunlit surface waters of the oceans are highly productive, and most of the carbon fixed in photosynthesis is remineralized by bacteria and other microorganisms in the upper ocean [43] . A small fraction of the organic carbon utilized by bacteria escapes rapid remineralization and appears as a slowly cycling reservoir of dissolved molecules of great chemical complexity. The microbial carbon pump concept suggests that the ‘successive—and perhaps repetitive—processing’ of labile DOM leads to the formation of refractory DOM [3] , [4] . The results from this study emphasize that exometabolites that are directly released by bacteria during the utilization of labile substrates could have intrinsic properties rendering them resistant to decomposition. The bacterial production of chemically complex and slowly cycling metabolites that accumulate in marine DOM occurs on much shorter time scales than those of ocean mixing [44] . Hence, the production of these persistent molecules is expected to closely reflect changes in primary production, and the efficacy of carbon sequestration by marine bacteria in the microbial carbon pump could be of similar magnitude as the particle flux to deep-sea sediments [45] . Disregarding DOM as a rapidly responding carbon reservoir biases model calculations of the oceanic capacity for atmospheric CO 2 sequestration. Systemic approaches are needed to understand the complex biological interactions regulating carbon fixation, remineralization and sequestration in the ocean. The imbalance between the biological processes of carbon fixation and remineralization has controlled carbon sequestration and shaped the composition of the atmosphere throughout the history of life on Earth. Bacteria are key drivers of these processes, and it appears they also play a major role in carbon sequestration through the production of diverse and complex dissolved molecules that can persist for millennia. Bioassay experiments setup Acid-cleaned 50 l carboys (high-density polyethylene (HDPE), Nalgene) were used to set up the bioassay experiments. All glasswares were combusted (400 °C, 4 h) and Milli-Q water (MQW, 18 MΩ, Millipore EliX 5 with Milli-Q Advantage A10 and ultraviolet) was used. In each carboy, ~42 l artificial sea water using precombusted anhydrous salts (NaCl, MgSO 4 , MgCl 2 , CaCl 2 , KCl, KBr and NaF; 400 °C, 4 h) and H 3 BO 3 and NaHCO 3 was added [46] . The salinity and the pH (adjusted with 2 mol l −1 HCl, ACS grade, Fisher Scientific) matched those of the coastal sea water at the site of the microbial inoculum collection (Folly Beach, South Carolina, USA). Before adding the substrate compounds and the inoculum, the artificial sea water was saturated with oxygen, and organic carbon in the carboys was below the detection limit. In one carboy, glucose (189 mg) and glutamic acid (185 mg) monomers were added as easily utilizable substrates (‘monomers’: 283 μmol C l −1 ). In the second carboy, cellobiose disaccharide (111 mg), stachyose tetrasaccharide (50 mg), Val-tyr-val tripeptide (98 mg), Leu-enkephalin pentapeptide (10 mg) and angiotensin octapeptide (1 mg) were combined (‘oligomers’: 269 μmol C l −1 ) to mimic a more diverse and complex substrate thereby stimulating the expression of specific hydrolytic enzymes by the microbial community. The substrate mixtures and inorganic nitrogen and phosphorus (106C:16N:1P molar ratio) were dissolved in MQW and mixed into the artificial sea water immediately before adding the microbial inoculum. Coastal sea water was collected below the surface microlayer (acid-cleaned 10 l HDPE carboy) and was filtered with combusted glass fibre filters (1.5 μm, Whatman 934-AH, 400 °C, 4 h) to remove larger particles and plankton. The microbial inoculum was further concentrated (nominal factor: 4.2) on a filter (0.2 μm, Supor, Millipore) and the supernatant decanted. A 50 ml volume of this solution was mixed into each carboy resulting in a dilution factor of 200 v/v for the microbial inoculum and 840 v/v for the coastal DOM. The time between coastal seawater collection and start of the bioassay experiments was <10 h. The contribution of dissolved organic carbon (DOC) from coastal sea water was <0.2 μmol l −1 in the bioassay carboys. The carboys were incubated at room temperature (21–26 °C) in the dark. At the end of the bioassay experiment (day 29), the water in the carboys was filtered (0.2 μm cartridge, Nuclepore, prerinsed with 10 l MQW) into an acid-cleaned HDPE carboy. All samples for further analysis were taken from this filtrate. Extraction of DOM Solid-phase extraction was performed using standard methods [47] . Briefly, SPE cartridges (PPL, 5 g, Agilent) were rinsed with methanol (HPLC grade, Merck) and activated with MQW (pH 2, HCl ACS grade, Fisher Scientific). The filtrates were acidified (pH 2) and extraction was conducted at a flow rate of 20 ml min −1 using a peristaltic pump in suction configuration. The cartridges were extensively rinsed with MQW (pH 2) and completely dried with N 2 before elution with methanol (25 ml). Coastal sea water (0.2 μm filtrate from inoculum enrichment) was extracted for reference DOM measurements. A process blank including substrate was prepared and this background DOC was 0.33 μmol l −1 in the carboys. The extraction efficiency (total DOC recovered from SPE cartridges) was 49 and 54% for the bacterial DOM and 80% for the coastal seawater DOM. Extracts were dried and stored under a N 2 atmosphere. Microbial cell enumeration Abundances of bacteria and heterotrophic nanoflagellates were determined by epifluorescence microscopy using the DAPI (4′,6-diamidino-2-phenylindole) method [10] . Water samples (0.5–2 ml) were stained with DAPI and filtered onto black-stained polycarbonate filters (0.2 μm, Millipore) mounted on prewetted cellulose filters (0.45 μm, Nuclepore). Twenty grid fields per sample were enumerated for bacteria and nanoflagellates (relative s.d. (r.s.d. ): ±15%). The occurrence of nanoflagellate grazers was first noted on days 9 and 10 in the monomer and oligomer experiments, respectively. Organic carbon and amino acid analysis Concentrations of total organic carbon (TOC) and DOC in unfiltered and filtered (0.2 μm, Supor, Whatman) water, respectively, was measured using a Shimadzu TOC-V CSN +TN. Reported concentrations were blank corrected, and instrument performance was evaluated daily with a deep-ocean reference standard [10] . Particulate organic carbon (r.s.d. : ±10%) was calculated as the difference between TOC and DOC (r.s.d. : ±5%) samples. The DOC concentration in SPE extracts was measured with a manual injector after evaporation of methanol (50 μl) with N 2 , dissolving with 0.6 ml MQW (pH 2) and purging with Ar for >5 min. Total dissolved hydrolysable amino acid (TDAA) concentrations were determined using HPLC and racemization correction [11] . Bioassay samples were filtered (0.2 μm, Supor), hydrolysed with 6 mol l −1 HCl (ACS plus, BDH) and separated on a Poroshell 120 EC-C18 column (4.6 × 100 mm, 2.7 μm, Agilent) after derivatization with o -phthaldialdehyde and N -isobutyryl- L -cysteine. TDAA comprised 18 amino acids: L - and D -alanine ( L- Ala, D- Ala), β-alanine, γ-aminobutyric acid, L- arginine, L - and D -asparagine+aspartic acid ( L- Asx, D- Asx), L - and D -glutamine+glutamic acid ( L- Glx, D- Glx), L- histidine, L- leucine, L- phenylalanine, glycine, L - and D -serine, L- threonine, L- tyrosine and L- valine (TDAA r.s.d. : ±15%). The D and L enantiomers of three pairs of amino acids were quantified (Ala, Asx and Glx) and expressed as the D/L ratio of the combined concentrations (D/L r.s.d. : ±15%). FT–ICR mass spectrometry analysis Dried DOM extracts were dissolved in methanol/MQW (1:1, v/v) to yield 0.8 mmol l −1 DOC and analysed with a Fourier transform ion cyclotron resonance (FT-ICR) mass spectrometer (solariX XR, Bruker Daltonics Inc., Billerica, MA) equipped with a dynamically harmonized analyser cell and a 12-T refrigerated actively shielded superconducting magnet (Bruker Biospin, Wissembourg, France). An electrospray ionization source was used in negative ion mode (capillary voltage: +4.5 kV) with a syringe pump for continuous infusion of the sample (2 μl min −1 ) and 200 single scans were added for acquisition of each mass spectrum. FT–ICR mass spectra were externally calibrated with arginine cluster and internally recalibrated with compounds that were repeatedly found in DOM samples [22] and the average mass error of the calibration mass peaks was 45±5 p.p.b. All mass peaks were singly charged ions (confirmed by the spacing of high magnitude 12 C x and 13 C 12 C x−1 peaks) and the m/z ratio represents (molecular) mass (Da) of the molecules. Molecular formulas (MFs) were calculated from masses in the range of 150–650 Da with an accuracy ≤±500 p.p.b. with a home-built algorithm, allowing for the following elemental compositions: 12 C 1-60 13 C 0-1 H 0-122 O 0-40 N 0-3 32 S 0-2 34 S 0-1 P 0-1 . For unambiguous elemental formula assignment the ‘nitrogen-rule’ and elemental ratios O/C≤1, N/C≤1, H≤2C+2+N (refs 12 , 48 ) were applied. Corresponding 13 C or 34 S isotope mass peak magnitudes were used for verification of the MF for high magnitude peaks. Remaining ambiguously assigned mass peaks were checked with the chemical building block approach [48] . Using FT–ICR mass spectrometry, no information about the structure can be obtained, hence a MF of a mass peak is only referred to as ‘molecule’ in this article. All samples (bacterial DOM from two bioassay experiments and coastal seawater DOM) were measured in duplicate. Root-mean-square error of mass accuracy of the calculated MF in the entire data set ( n =6 samples) was 170 p.p.b. Peak repeatability was 74% for bacterial DOM and 86% for the coastal seawater DOM. MFs in the process blank were excluded from all samples. Less than 4% of the carbon in the bacterial DOM extracts could potentially derive from the coastal seawater DOM. A standard addition (bacterial DOM spiked with increasing amounts of coastal seawater DOM) was carried out to identify and exclude mass peaks in the bioassay DOM that were exclusively derived from the coastal seawater DOM. These peaks were identified based on their intensity correlation with the added coastal DOM and the conservative estimate of coastal DOM (0.2 μmol C l −1 ) initially introduced with the inoculum (resulting in exclusion of 165 peaks or <2% of total intensity in bacterial DOM spectra). Hence corrected bacterial DOM spectra only contained mass peaks from molecules produced during the bioassay experiment. For the duplicate measurements, mass peaks with a signal-to-noise ratio (S/N) >6 in one replicate and at least >4 in the second replicate were used to obtain an average mass spectrum for each sample (relative reproducibility of mass peak intensity >93%). Relative intensities of each mass peak in the data set were calculated from the sum of all mass peaks (=100% intensity). Overall, this most conservative approach resulted in 1,717 and 1,796 MFs for the bacterial DOM samples and 3,036 MF for the coastal seawater DOM. The molecular double bond equivalent (DBE) was calculated as: DBE=1+½(2C−H+N+P) where C, H, N and P are the number of carbon, hydrogen, nitrogen and phosphorus atoms in a molecular formula. CRAM are a broadly defined class of molecules and were identified by their molecular ratios DBE/C (0.30–0.68), DBE/H (0.20–0.95) and DBE/O (0.77–1.75) (ref. 18 ). NMR analysis Proton NMR spectra ( noesypr1d ) of solid-phase extracted DOM were acquired immediately after sample preparation in CD 3 OD (99.95% 2 H, Aldrich, Steinheim) with a Bruker Avance III NMR spectrometer operating at 800.13 MHz (B 0 =18.8 T) with an inverse geometry 5 mm z-gradient quaternary 1 H/ 13 C/ 15 N/ 31 P QCI cryogenic probe (quaternary cryogenic inverse; 90° excitation pulses: 13 C~ 1 H~10 μs). The one-dimensional 13 C NMR spectra were acquired in 12 CD 3 OD solution (<0.05% 13 C, Aldrich, Steinheim) at 125.77 MHz (B 0 =11.7 T) with a 5 mm z-gradient dual 13 C/ 1 H cryogenic probe (90° excitation pulses: 13 C~11 μs and 1 H~17 μs) with a total acquisition time of >10 days for each sample. Two-dimensional, carbon decoupled, 1 H, 13 C DEPT HSQC (distortionless enhanced polarization transfer heteronuclear single quantum coherence: hsqcetgpsisp2.2 ) spectra were acquired at 800.13 MHz with 256/320 scans (F2, 1 H) and 800/640 increments with a carbon sweep width of 210 p.p.m. (F1, 13 C). Data were computed on an 8,192 × 1,024 matrix with shifted sine bell in F1 and exponential line broadening in F2. The NMR chemical shift references were: 1 H NMR, HD 2 COD: 3.30 p.p.m. ; 13 C NMR, CD 3 OD: 49.00 p.p.m. All spectra were acquired with TopSpin 3.2/PL3 software at 283 K; acquisition parameters closely followed those used in ref. 13 and are depicted in Supplementary Table 1 . Proton and carbon NMR key substructures (sections) were defined according to ref. 13 and 1 H and 13 C spectra were integrated with a bucket width of 0.01/1 p.p.m. (AMIX, ver. 3.9.4) to compute NMR section integrals. CH 2 -selective 1 H, 13 C NMR spectra were colour coded for CH 3 (red) and CH 2 (green). Manual coloration was applied for methine carbon (CH: brown) and noise (bright grey) with consideration of methoxy (OCH 3 ) cross peaks (red, δ ( 13 C): 48–64 p.p.m. ; δ ( 1 H): 5–3.2 p.p.m.) from CH 3 -selective 1 H, 13 C DEPT HSQC NMR spectra. The sample amounts (dry weight) used for the NMR analyses were 5.7 and 4.9 mg for the ‘monomer’ and ‘oligomer’ experiments, respectively, and 36.2 mg for DOM from East Atlantic surface water (48 m depth, cf . ref. 13 ). How to cite this article: Lechtenfeld, O. J. et al . Marine sequestration of carbon in bacterial metabolites. Nat. Commun. 6:6711 doi: 10.1038/ncomms7711 (2015).